Water clustering on nanostructured iron oxide films The adhesion of water to solid surfaces is characterized by the tendency to balance competing molecule–molecule and molecule–surface interactions. Hydroxyl groups form strong hydrogen bonds to water molecules and are known to substantially influence the wetting behaviour of oxide surfaces, but it is not well-understood how these hydroxyl groups and their distribution on a surface affect the molecular-scale structure at the interface. Here we report a study of water clustering on a moiré-structured iron oxide thin film with a controlled density of hydroxyl groups. While large amorphous monolayer islands form on the bare film, the hydroxylated iron oxide film acts as a hydrophilic nanotemplate, causing the formation of a regular array of ice-like hexameric nanoclusters. The formation of this ordered phase is localized at the nanometre scale; with increasing water coverage, ordered and amorphous water are found to coexist at adjacent hydroxylated and hydroxyl-free domains of the moiré structure. Motivated by applications in diverse fields such as electrochemistry, geochemistry, atmospheric chemistry, corrosion and catalysis, the structure of water adsorbed on solid surfaces has been a topic of strong and sustained interest over the past decades [1] , [2] , [3] , [4] . Due to the relative strength and particular directionality of interactions between water molecules, which are delicately balanced against molecule–surface interactions, the structures of water monolayers on various surfaces exhibit surprising diversity. This has been recently demonstrated in scanning tunnelling microscopy (STM) studies [5] , [6] , [7] , [8] , which allow direct visualization of hydrogen bonding networks. The most detailed insight into water adsorption has been achieved for single-crystal metal surfaces, where the structure of water layers is determined mainly by the dimensions of the surface unit cell and the strength of metal–oxygen bonding [6] . The adsorption and clustering of water on metal oxide surfaces are very relevant for applications, as these materials are ubiquitous under ambient and aqueous conditions. Oxides add an additional level of complexity compared with metals, as water molecules can bond both to metal cations and oxide anions, and in addition, adhere strongly to OH groups formed by water dissociation at lattice sites or at abundant structural defects [3] , [9] , [10] , [11] , [12] , [13] , [14] , [15] , [16] , [17] . Although these fundamental aspects of water adsorption on oxide surfaces have been well-established, comparatively few microscopy studies have been conducted to provide detailed information about the structures formed and the influence of defects. As a result, understanding of water adsorption on oxides remains far behind that of adsorption on metals. An additional relevant factor in the adsorption of water on the surfaces of natural or man-made materials is the fact that many such materials have nanometre-scale dimensions, and thus present an adsorption landscape for water which is inhomogeneous. Such inhomogeneity can lead to the formation of distinct nanometre-scale water structures, as observed on a boron nitride nanomesh [18] , or can disrupt the formation of an ordered phase, as observed on stepped Pt surfaces [19] . On oxide surfaces, an inhomogeneous distribution of defects or the presence of different facets can lead to a strongly varying distribution of OH groups, creating large variations in hydrophilicity over short length scales [16] . In general it is not well-understood how nanoscale variations in surface structure impact the formation and structure of the first few wetting layers on oxide surfaces. Monolayer FeO grown on Pt(111), first reported by Vurens et al. [20] , exhibits a 2.5 nm moiré superstructure due to the ~10% lattice mismatch between the FeO film and the substrate [21] . The resulting modulation in the film’s structure, best understood in terms of periodic variation in Fe-O buckling normal to the surface, creates an inhomogeneous adsorption potential [22] , so that adsorbed atoms and molecules have been found to form arrays with the periodicity of the film’s superstructure instead of forming larger, more random aggregates [23] , [24] . Although previous temperature-programmed desorption (TPD), infrared reflection absorption spectroscopy and ultraviolet photoelectron spectroscopy studies of water adsorbed on ultra-thin FeO(111) films have shown rather weak interactions between water and the surface [12] , [25] , [26] , no microscopy studies have been reported to date and the potential effect of the films’ moiré structure on the adsorption has not been considered. Additionally, as demonstrated in previous studies [27] , [28] , [29] , OH groups can be introduced to the FeO surface in a well-controlled manner by exposure to atomic hydrogen, enabling us to directly and systematically study the effects of hydroxylation on H 2 O adsorption and clustering. As will be discussed below, the OH groups formed in this manner also show a distinct spatial distribution following the film’s moiré structure, allowing us to examine the impact of nanometre-scale variations in defect density. We report here a combined experimental and theoretical study of water adsorption, clustering and desorption on bare and hydroxylated monolayer FeO/Pt(111) at low temperatures. Our results show that hydroxyl groups on the FeO film promote the formation of an ordered, ice-like phase, in contrast to the disordered structure formed on the bare surface. The OH groups are localized at one particular domain of the FeO film’s moiré unit cell, such that the surface exhibits alternating hydrophilic and hydrophobic regions with a periodicity of ~2.5 nm. Despite the small length scale, it is found that the ordered phase only forms at the hydrophilic domains—not at adjacent hydrophobic domains. Hydroxylation of FeO with atomic hydrogen An STM image of the bare FeO/Pt(111) surface is displayed in Fig. 1a , with a structural model of the film shown in Fig. 1b . As is clear in the STM image, the FeO film exhibits a distinct moiré superstructure, which can be described in terms of three high-symmetry domains. These domains are distinguished by the local stacking sequence of the Fe and O layers relative to the high-symmetry points of the Pt(111) surface. At the FCC domain (square), Fe ions reside above fcc hollow sites and O ions reside above hcp hollow sites; at the HCP domain (triangle), Fe ions reside above hcp hollow sites and O ions reside above Pt atoms; at TOP domains (circle), Fe ions reside above Pt atoms and O ions reside above fcc hollow sites. Unambiguous identification of the different domains in STM images has been achieved through intentional creation of defects in the FeO film [30] , [31] . It has been shown that, under the imaging conditions of Fig. 1a , the bright points in the TOP domains correspond to Fe ions while the bright points at the FCC domains correspond to O ions [30] . 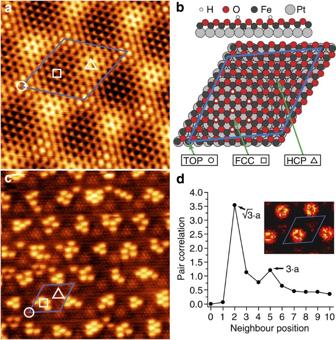Figure 1: Bare and hydroxylated FeO films. (a) STM image of the bare FeO/Pt(111) film (65 × 65 Å2, 65 mV, 3 nA). The moiré unit cell and high-symmetry domains are indicated. Circle, square, and triangle are used to denote TOP, FCC and HCP domains, respectively. (b) Ball model of the FeO/Pt(111) film. The ~25 Å moiré unit cell is indicated as are the three high-symmetry domains. OH groups are shown (with white dots for H atoms) in the preferred FCC domain of the moiré unit cell in their preferred (√3 × √3) R30° arrangement. (c) STM image (140 × 140 Å2, 0.7 V, 0.4 nA) of the hydroxylated FeO film with an OH coverage of 0.05 ML, acquired at 160 K after additionally dosing ~0.02 ML water (not visible). (d) Pair correlation function for OH groups showing peaks at the second nearest neighbour and fifth nearest neighbour positions, indicating local (√3 × √3) R30° ordering. Inset: distribution of OH groups within the moiré cell, showing the preference for occupation of FCC domains. Figure 1: Bare and hydroxylated FeO films. ( a ) STM image of the bare FeO/Pt(111) film (65 × 65 Å 2 , 65 mV, 3 nA). The moiré unit cell and high-symmetry domains are indicated. Circle, square, and triangle are used to denote TOP, FCC and HCP domains, respectively. ( b ) Ball model of the FeO/Pt(111) film. The ~25 Å moiré unit cell is indicated as are the three high-symmetry domains. OH groups are shown (with white dots for H atoms) in the preferred FCC domain of the moiré unit cell in their preferred (√3 × √3) R30° arrangement. ( c ) STM image (140 × 140 Å 2 , 0.7 V, 0.4 nA) of the hydroxylated FeO film with an OH coverage of 0.05 ML, acquired at 160 K after additionally dosing ~0.02 ML water (not visible). ( d ) Pair correlation function for OH groups showing peaks at the second nearest neighbour and fifth nearest neighbour positions, indicating local (√3 × √3) R30° ordering. Inset: distribution of OH groups within the moiré cell, showing the preference for occupation of FCC domains. Full size image Figure 1c shows an STM image of an FeO film which has been exposed to atomic hydrogen, leading to protonation of ~5% of the FeO lattice oxygen ions (see Fig. 1b ). Throughout this work we refer to these protonated O ions as hydroxyls or OH groups, and to the surface prepared in this way as being hydroxylated. The image in Fig. 1c was acquired at 160 K after additionally dosing ~0.02 monolayer (ML) water onto the surface to promote H atom mobility [29] , allowing equilibration of the structure, and to ensure that the effects of adsorbed water on the spatial distribution of OH groups are accounted for. This results in a more well-ordered distribution compared with what is observed directly after H atom exposure (see Supplementary Fig. 1 ). The OH groups appear in STM images as bright protrusions [31] , and due to rapid diffusion at this temperature, the coadsorbed H 2 O is not visible. From the distribution of OH groups relative to the moiré structure ( Fig. 1d , inset), we find a strong preference for occupation of FCC domains, followed by partial occupation of HCP domains. The local arrangement of OH groups is also not random, as evidenced by their pair correlation function extracted from this image, plotted in Fig. 1d . Here the prominent peak at the second-nearest-neighbour position (corresponding to a separation of √3· a , where a is the 3.1 Å FeO lattice parameter) and smaller peak at the fifth-nearest-neighbour position (corresponding to a separation of 3· a ) indicate a strong tendency towards local (√3 × √3) R30° ordering. Such an arrangement is depicted in Fig. 1b . Density functional theory (DFT) calculations show that the (√3 × √3) R30° ordering results essentially from repulsion between neighbouring OH groups; the binding energy of a single H atom in the FCC domain is −2.75 eV, while the differential binding energy of a second H atom at a nearest-neighbour site is −2.65 eV and at a second-nearest-neighbour site is −2.73 eV. Thus, the second hydroxyl at the second-nearest-neighbour site is 0.08 eV more stable than that in the nearest-neighbour configuration. 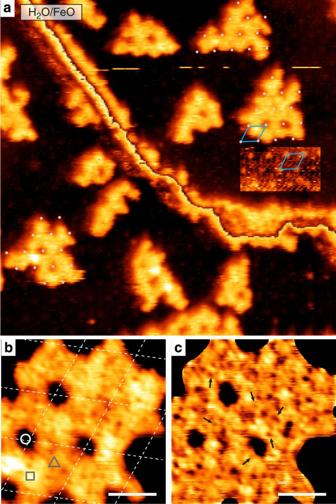Figure 2: Water adsorption on bare FeO. (a) STM image (480 × 480 Å2) of water adsorbed on the bare FeO/Pt(111) film, acquired at 110 K. The moiré unit cell is indicated in blue and the positions of TOP domains in the vicinity of three H2O islands are indicated with grey dots. The rectangular area shows enhanced contrast of the bare FeO film, where bright spots are seen corresponding to the TOP domains. The image shows two terraces (higher terrace in the upper right) separated by a single-atomic-height step in the Pt(111) substrate. A cyclic colour scale is used to improve contrast. (b) High-magnification STM image of a H2O island on the bare FeO film. This image is the average of four successive STM measurements at 110 K. The grid marks the moiré unit cells, and the different domains are labelled as inFig. 1b. Scale bar, 20 Å. (c) The same STM image as inbafter subtraction of the long-range height variations. Arrows indicate some of the 4–5 Å pores observed in the structure. Scale bar, 20 Å. Effect of hydroxylation on water clustering Figure 2a shows an STM image of water on bare FeO at 110 K, following exposure at ~130 K. Adsorbed water forms two-dimensional islands on the terraces and elongated clusters along the step edges. The irregular shapes of the water islands on the terraces result from the moiré structure, with voids formed preferentially at one type of domain, appearing brightest in the STM image (see contrast-enhanced inset in Fig. 2a ), several of which are marked with grey dots. Under the imaging conditions employed here (+1.4 V, 0.2 nA), these bright regions in STM images of the bare FeO film correspond to TOP domains [30] where Fe ions occupy sites above Pt atoms. The tendency of water to avoid wetting these domains is an indication that interactions between water molecules and Fe ions play no significant role in the structure; we find by DFT calculations that water monomers adsorb most strongly (−0.21 eV adsorption energy) at Fe sites of TOP domains, where a larger in-plane atomic spacing and smaller Fe-O rumpling make these cations more easily accessible compared with the FCC and HCP domains, where monomer adsorption energies of −0.11 and −0.13 eV were calculated. The strong preference for water to occupy FCC and HCP domains rather than TOP domains is therefore attributed to the significantly weaker electrostatic field above O atoms at TOP domains caused by the smaller rumpling of the FeO [22] , [32] , [33] . Figure 2: Water adsorption on bare FeO. ( a ) STM image (480 × 480 Å 2 ) of water adsorbed on the bare FeO/Pt(111) film, acquired at 110 K. The moiré unit cell is indicated in blue and the positions of TOP domains in the vicinity of three H 2 O islands are indicated with grey dots. The rectangular area shows enhanced contrast of the bare FeO film, where bright spots are seen corresponding to the TOP domains. The image shows two terraces (higher terrace in the upper right) separated by a single-atomic-height step in the Pt(111) substrate. A cyclic colour scale is used to improve contrast. ( b ) High-magnification STM image of a H 2 O island on the bare FeO film. This image is the average of four successive STM measurements at 110 K. The grid marks the moiré unit cells, and the different domains are labelled as in Fig. 1b . Scale bar, 20 Å. ( c ) The same STM image as in b after subtraction of the long-range height variations. Arrows indicate some of the 4–5 Å pores observed in the structure. Scale bar, 20 Å. Full size image A high-resolution STM image of one water island on the bare FeO film is shown in Fig. 2b . Despite some enhanced noise in such images, suggesting possible diffusion of the molecules or interactions with the STM tip, sequential images of the same island acquired over a period of ~2 min show the structure to be essentially static (see Supplementary Fig. 2 ). To increase the signal-to-noise ratio, four sequentially-acquired STM images were averaged to obtain the image shown in Fig. 2b . To further enhance the molecular-scale contrast, we removed the long-range variation in apparent height of the water layer by subtraction of a polynomial background (see Supplementary Fig. 3 ), and the result is displayed in Fig. 2c . Although individual water molecules are not resolved, the image clearly shows an absence of crystalline order, indicating the formation of an amorphous hydrogen-bonded network. Several pores are discernible with diameters in the range of 4–5 Å, some of which are indicated in Fig. 2c . These pores arise from ring structures incorporating roughly 5–6 H 2 O molecules, similar to those observed in ordered structures on metal surfaces [4] , [5] . The apparent height of the water layer varies between the different domains of the FeO moiré structure. Considering the very weak chemical interactions between the molecules and the surface, these differences may indicate variations in the height of the water layer above the FeO film. According to DFT calculations [30] the heights of the FeO oxygen ions above the Pt interface layer follow the order TOP (307 pm)>FCC (304 pm)>HCP (298 pm), whereas the apparent height of the water layer above the FCC domains is consistently larger than that over the HCP domains and the single occupied TOP domain by 15–30 pm. This observation is consistent with the stronger electrostatic field at the FCC domains, causing a greater tendency towards vertical orientation of the water molecules, with O–H bonds directed towards the surface [34] . The presence of surface hydroxyls on the FeO film, introduced using atomic hydrogen, changes the adsorption behaviour of water entirely, as demonstrated in Fig. 3a . Here instead of extended islands, we observe small, separated water clusters confined to the FCC domains of the moiré unit cells. Thus, the strong affinity of water for surface OH groups enables the FeO film, which itself exhibits a relatively flat potential energy surface for water adsorption, to act as a nanoscale template for water clusters. 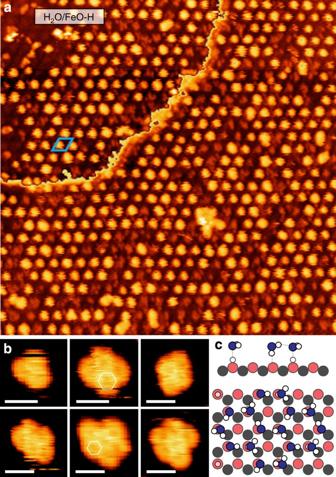Figure 3: Water adsorption on hydroxylated FeO. (a) STM image (600 × 600 Å2) of water adsorbed on a hydroxylated FeO film with an OH coverage of 0.05 ML, acquired at 110 K. The moiré unit cell is indicated in blue. The image shows two terraces (higher terrace in the upper left) separated by a single-atomic-height step in the Pt(111) substrate. A cyclic colour scale is used to improve contrast. (b) High-magnification images of H2O clusters on hydroxylated FeO showing a hexagonal ring structure. Scale bars, 10 Å. (c) Schematic model of the hexagonal ring structure on hydroxylated FeO inferred from STM measurements; upper section gives a cross-section view; bottom an atop view. Figure 3: Water adsorption on hydroxylated FeO. ( a ) STM image (600 × 600 Å 2 ) of water adsorbed on a hydroxylated FeO film with an OH coverage of 0.05 ML, acquired at 110 K. The moiré unit cell is indicated in blue. The image shows two terraces (higher terrace in the upper left) separated by a single-atomic-height step in the Pt(111) substrate. A cyclic colour scale is used to improve contrast. ( b ) High-magnification images of H 2 O clusters on hydroxylated FeO showing a hexagonal ring structure. Scale bars, 10 Å. ( c ) Schematic model of the hexagonal ring structure on hydroxylated FeO inferred from STM measurements; upper section gives a cross-section view; bottom an atop view. Full size image In addition to altering the size and shape of water clusters formed on FeO, the presence of OH groups has a striking effect on the molecular-scale ordering of the water within the clusters. Figure 3b shows high-magnification STM images of H 2 O clusters of various sizes observed on a hydroxylated FeO film. The clusters exhibit a distinct hexagonal ring motif with apparent (√3 × √3) R30° symmetry, similar to ring structures that have been observed on several metal surfaces [2] . Assuming that the preferential (√3 × √3) R30° ordering of OH groups observed on FeO ( Fig. 1c,d ) is retained upon exposure to water, half of the H 2 O molecules in the hexagonal structure should lie flat, accepting hydrogen bonds from the surface OH while the other half should be oriented vertically, donating hydrogen bonds to surface O ions. A schematic model of the proposed structure is depicted in Fig. 3c . DFT calculations of water clusters on FeO To gain further insight into the water structures observed on the hydroxylated surface, we carried out DFT+U calculations using, for simplicity, a single cyclic water hexamer [35] , [36] adsorbed at the FCC domain of the FeO film populated with OH groups arranged in a (√3 × √3) R30° pattern (see Fig. 1b ). The cyclic hexamer is the basic structural motif of ice I h . The most stable isomer in the gas phase has S 6 symmetry and each H 2 O molecule simultaneously acts as a H-bond donor and acceptor ( Supplementary Fig. 4 ). The relaxed, lowest-energy structure of an S 6 -like water hexamer adsorbed onto hydroxylated FeO, whose symmetry is reduced upon adsorption to that of point group C 3 , is depicted in Fig. 4a,b . Three of the six H 2 O molecules are oriented parallel to the surface, accepting hydrogen bonds from the surface OH (green dashed lines in Fig. 4a ), and the remaining three H 2 O molecules are oriented perpendicular to the surface, with one O–H bond oriented downwards towards a surface O atom (white dashed lines in Fig. 4a ). 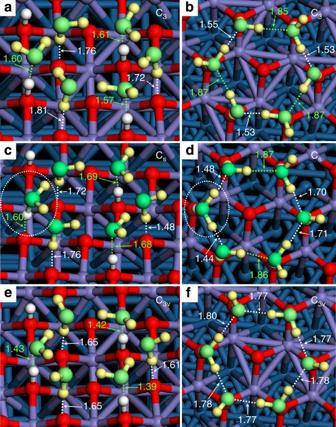Figure 4: Atomic structures of water clusters on hydroxylated FeO. Tilted side (a,c,e) and top (b,d,f) views of three cyclic water hexamers, differing in the orientations of the molecules, adsorbed on the hydroxylated FeO film as determined by DFT+U calculations. All numerical values for bond lengths are in Å. Green (white) dashed lines ina,c,eindicate hydrogen bonds between the hexamer and the surface where the water acts as a hydrogen bond acceptor (donor). Green (white) dashed lines inb,d,findicate hydrogen bonds where the parallel water is accepting (donating) a hydrogen bond. Note the transfer of one H+ion from the surface to one water molecule, forming a hydronium (H3O+) ion, in theCsstructure, highlighted by dashed white ovals inc,d. Blue, purple, red and white spheres indicate Pt, Fe, O and H atoms, respectively. H and O atoms in H2O are highlighted by yellow and green spheres, respectively. Figure 4: Atomic structures of water clusters on hydroxylated FeO. Tilted side ( a , c , e ) and top ( b , d , f ) views of three cyclic water hexamers, differing in the orientations of the molecules, adsorbed on the hydroxylated FeO film as determined by DFT+U calculations. All numerical values for bond lengths are in Å. Green (white) dashed lines in a , c , e indicate hydrogen bonds between the hexamer and the surface where the water acts as a hydrogen bond acceptor (donor). Green (white) dashed lines in b , d , f indicate hydrogen bonds where the parallel water is accepting (donating) a hydrogen bond. Note the transfer of one H + ion from the surface to one water molecule, forming a hydronium (H 3 O + ) ion, in the C s structure, highlighted by dashed white ovals in c , d . Blue, purple, red and white spheres indicate Pt, Fe, O and H atoms, respectively. H and O atoms in H 2 O are highlighted by yellow and green spheres, respectively. Full size image The hydrogen bonds inside the cyclic ring have two different general lengths, which alternate around the ring. This can be understood by focusing on one parallel-oriented water molecule: The accepted H-bond is longer (1.85–1.87 Å), whereas the donated H-bond is shorter (1.53–1.55 Å). Inside the cyclic ring the average length of H-bonds is 1.70 Å, slightly longer (by 0.05 Å) than that of a cyclic water hexamer in the gas phase ( Supplementary Fig. 4 ), due to the influence of hydrogen bonds with the surface. The H-bonds between the parallel H 2 O and surface OH are in the range of 1.57–1.61 Å, while the H-bonds between the perpendicular H 2 O and surface O are longer (1.72–1.81 Å). The parallel H 2 O molecules are slightly tilted relative to the surface, with an average vertical displacement of 0.35 Å between the two H in the parallel H 2 O. This displacement is smaller than the value for the S 6 hexamer in the gas phase (0.78 Å, projected along the S 6 axis). The average adsorption energy of H 2 O in the C 3 hexamer ( Fig. 4a,b ), relative to isolated, gas-phase H 2 O molecules, is calculated to be −0.68 eV per H 2 O. For reference, the adsorption energy of an isolated H 2 O molecule hydrogen bonded to a surface OH is −0.62 eV and that of an isolated molecule on the bare FeO surface ranges from −0.1 to −0.2 eV, depending on the moiré domain. H 2 O adsorbed as a C 3 hexamer on the bare FeO surface ( Supplementary Fig. 5 ) has a mean adsorption energy of −0.42 eV per H 2 O molecule (referenced to isolated gas-phase H 2 O), nearly all of which is due to intermolecular hydrogen bonding; for a similar S 6 cyclic hexamer in the gas phase ( Supplementary Fig. 4 ) we calculate a formation energy of −0.39 eV per H 2 O. In bulk ice I h , where all H 2 O molecules are found in a tetrahedral bonding arrangement, each donating and accepting two hydrogen bonds to its neighbours, the positions of the protons (that is, the orientations of the water molecules) do not exhibit crystalline order but are instead random, within the constraint that the H-bonds remain saturated, and a transition to an ordered structure only occurs at very low temperatures [37] . Breaking of the bulk symmetry, as occurs at surfaces and in nanostructures, has the potential to induce proton ordering by eliminating the near-degeneracy of structures with water molecules in different orientations [38] , [39] . To investigate the extent of proton ordering in H 2 O nanoclusters on FeO, we performed additional calculations using a different cyclic hexamer where one of the H 2 O molecules acts as a double H-bond donor, and a second acts as a double H-bond acceptor ( Fig. 4c,d ). This cyclic H 2 O hexamer has C s symmetry and is 0.89 eV less stable in the gas phase than the S 6 hexamer discussed above. Remarkably, when adsorbed on hydroxylated FeO, the C s hexamer is nearly isoenergetic with the adsorbed C 3 hexamer; the calculated average adsorption energy is −0.66 eV per H 2 O. A third hexamer, characterized by C 3v symmetry, with three double H-bond donors and three double H-bond acceptors ( Fig. 4e,f ), was likewise similar in energy to the adsorbed C 3 and C s hexamers; although unstable in the gas-phase calculation (it converged to the S 6 structure), on hydroxylated FeO the adsorption energy was calculated as −0.67 eV per H 2 O. Although the differences in energy between these configurations are too small to predict which will be dominant in experimentally-observable H 2 O clusters [40] , [41] , it is clear that the hydroxylated FeO surface significantly stabilizes bonding configurations that otherwise are unfavourable. This very likely leads to a significantly greater degree of proton disorder than would be expected based on gas-phase results. In the gas phase, the striking differences in stability of the three different cyclic hexamers result from the cooperative nature of hydrogen bonds in water [42] , [43] . Formation of a hydrogen bond between water molecules involves a polarization of each molecule’s electronic charge density towards the region between the two molecules where the hydrogen bond is formed. This polarization depletes electronic charge from the covalent O-H bonds of the acceptor molecule, increasing its tendency to act as a donor to another H 2 O molecule, which in turn experiences a similar polarization, and so on. The result is, depending on the configuration, an enhancement or diminishment in mean hydrogen bond strength compared with what would be expected based on pairwise interactions, that is, that observed in an H 2 O dimer. In the S 6 water hexamer, the position of each molecule as a simultaneous H-bond donor and acceptor takes full advantage of these effects and a corresponding increase in stability is observed. In the C s and C 3v hexamers, however, molecules are found which either donate two hydrogen bonds without accepting any, or which accept two hydrogen bonds without donating any. This unfavourable configuration leads to a reduction in hydrogen bond strength, significantly destabilizing the structures. However, by interaction with the hydroxylated FeO surface such effects are almost fully compensated. In the C 3v structure ( Fig. 4e,f ), the three double-donor H 2 O molecules accept strong hydrogen bonds from surface OH groups, with calculated O–H distances of 1.39–1.43 Å, while the three double-acceptor H 2 O molecules donate relatively strong bonds to the substrate O ions, with calculated O–H distances of 1.61–1.65 Å. The effects are even more pronounced for the C s isomer, where polarization of the double-donor H 2 O molecule is sufficient to draw the OH proton away from the surface, spontaneously forming an H 3 O + ion (indicated by the dashed oval in Fig. 4c,d ). The double-acceptor H 2 O at the opposite side of the molecule likewise interacts strongly with the surface, with a calculated O–H distance of 1.48 Å. Cooperative effects are also apparent in the adhesion of the C 3 hexamer ( Fig. 4a,b ). The weak interaction between the hexamer and the bare FeO surface is reflected in the H-bond lengths of the molecules with OH bonds directed towards the surface, which are calculated to be 2.06–2.07 Å (see Supplementary Fig. 5 ). The strong hydrogen bonds formed at surface OH groups on hydroxylated FeO impart substantial donor character to the associated flat-lying H 2 O molecules, which then form strong donor bonds to the neighbouring vertical H 2 O molecules, as reflected by the alternating bond lengths around the ring mentioned above. As a secondary effect, the acceptance of this strong H-bond by the vertically-oriented H 2 O molecules leads to a significant contraction of the hydrogen bond lengths between these molecules and the surface O ions, to 1.72–1.81 Å. Even for the FeO film, which should be considered a rather acidic oxide (on the basis of the relative strengths of donor and acceptor H-bonds with water [44] ), O ions adjacent to OH groups act as H-bond acceptors as a result of cooperative hydrogen bonding. These interactions effectively separate the hexamer into three associated dimers, each held together by an especially strong hydrogen bond (1.53–1.55 Å), qualitatively similar to what has been observed for water on TiO 2 (110) [17] and predicted for MgO(100) [45] and O/Ru(0001) [46] . The substantial donor character imparted to the ‘parallel’ H 2 O molecules by H-bonding to OH groups on hydroxylated FeO will create an effective repulsive interaction between these complexes, providing an additional driving force for the formation of a structure with (√3 × √3) R30° ordering of the underlying H atoms, independent of the intrinsic distribution of H atoms on the surface described above. A similar effect has been observed in mixed OH/H 2 O monolayers on Pt(111) (OH in this case referring to a distinct molecule coadsorbed with water), where very stable, ordered hexagonal structures form at a 1:1 (OH:H 2 O) ratio as a result of alternating H-bond donor (H 2 O) and acceptor (OH) molecules [47] , [48] . Such a tendency towards donor/acceptor ordering is expected to occur as a general feature of water adsorption on hydroxylated oxide surfaces, to the extent this is compatible with the geometric features of the specific surface. Desorption kinetics To investigate the effect of hydroxylation on the desorption behaviour of water, we conducted TPD measurements on the bare FeO film and on films with various OH coverages ( Fig. 5 ). For each surface, prepared initially by exposure of the FeO film to atomic hydrogen, H 2 O was dosed at 130 K and TPD traces were measured up to 250 K, after which the sample was re-cooled to 130 K and the next measurement was conducted. Reaction of OH groups to form H 2 O, leading to irreversible reduction of the surface, occurs only above ~400 K [28] . Similar to previous observations for a two-layer thick FeO(111) film [25] , the TPD traces from the bare film show a single peak (denoted α ) for sub-monolayer coverages at 164–168 K and an additional peak at ~158 K (denoted γ ) due to adsorption on top of the first wetting layer. On the hydroxylated FeO surface a new feature appears in the TPD spectra at higher temperatures, 167–186 K (denoted β ). With increasing OH coverage the β feature becomes more prominent and shifts to higher temperatures. As can be seen by comparing the traces plotted in red in Fig. 5a–e , growth of the β feature occurs at the expense of the α feature. 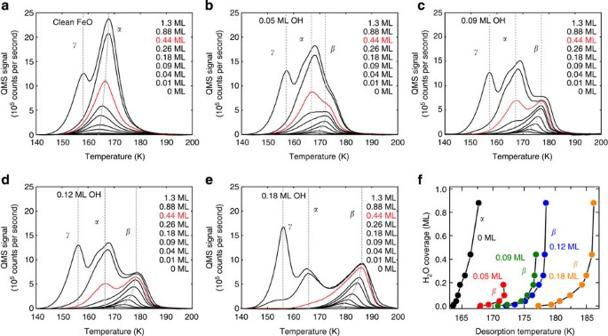Figure 5:Effect of hydroxylation on H2O desorption kinetics. TPD measurements (2 K s−1linear ramp) of H2O from (a) bare FeO/Pt(111), and hydroxylated FeO films with OH coverages of (b) 0.05 ML, (c) 0.09 ML, (d) 0.12 ML, (e) 0.18 ML. Dashed lines indicate primary desorption features (see text); traces obtained with an initial H2O coverage of 0.44 ML are plotted in red for easy comparison. (f) Plot of the peak temperature of the highest-temperature desorption feature (αfor bare FeO,βfor hydroxylated FeO) for various OH coverages and H2O exposures. Figure 5: Effect of hydroxylation on H 2 O desorption kinetics. TPD measurements (2 K s −1 linear ramp) of H 2 O from ( a ) bare FeO/Pt(111), and hydroxylated FeO films with OH coverages of ( b ) 0.05 ML, ( c ) 0.09 ML, ( d ) 0.12 ML, ( e ) 0.18 ML. Dashed lines indicate primary desorption features (see text); traces obtained with an initial H 2 O coverage of 0.44 ML are plotted in red for easy comparison. ( f ) Plot of the peak temperature of the highest-temperature desorption feature ( α for bare FeO, β for hydroxylated FeO) for various OH coverages and H 2 O exposures. Full size image Interpretation of the measured TPD traces is assisted by STM measurements of different quantities of water adsorbed on FeO surfaces with varying OH coverages. The STM images in Fig. 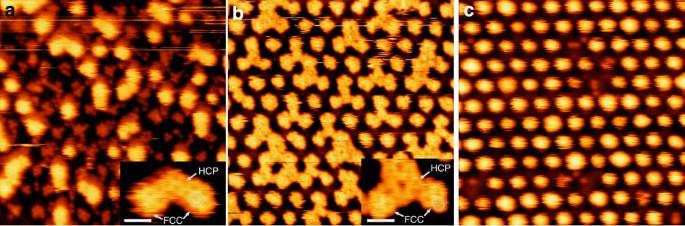Figure 6:Effects of OH and H2O coverages. STM images (250 × 250 Å2) of H2O adsorbed on hydroxylated FeO with various OH coverages and H2O exposures. (a) 0.1 ML H2O, 0.12 ML OH, (b) 0.25 ML H2O, 0.05 ML OH, (c) 0.1 ML H2O, 0.05 ML OH. Insets inaandbare high-resolution images of H2O clusters on the respective surfaces, showing the different structures at HCP domains with and without OH groups. Scale bars, 10 Å. 6 illustrate the effects of the relative H 2 O and OH coverages on the size and molecular structure of adsorbed water clusters at 110 K. Figure 6a,b shows surfaces where small and large quantities of water were dosed onto surfaces with high and low coverages of OH groups, respectively. On the surface ( Fig. 6a ) with an excess of OH groups, whose coverage is sufficient to populate HCP domains as well as FCC domains, we observed that the islands exhibit a clear hexagonal ring structure at both the FCC and HCP domains. In contrast, on the FeO surface with a low coverage of OH groups and an excess of water ( Fig. 6b ), the hexagonal ring structure is only observed at FCC domains; at the HCP domains, which are unoccupied by OH groups, a disordered structure is observed similar to that found on the bare FeO film. Figure 6: Effects of OH and H 2 O coverages. STM images (250 × 250 Å 2 ) of H 2 O adsorbed on hydroxylated FeO with various OH coverages and H 2 O exposures. ( a ) 0.1 ML H 2 O, 0.12 ML OH, ( b ) 0.25 ML H 2 O, 0.05 ML OH, ( c ) 0.1 ML H 2 O, 0.05 ML OH. Insets in a and b are high-resolution images of H 2 O clusters on the respective surfaces, showing the different structures at HCP domains with and without OH groups. Scale bars, 10 Å. Full size image Accordingly, under the conditions of the STM experiments, adsorbed water occurs in two distinct phases: an ordered phase associated with OH groups, and an amorphous phase associated with the bare FeO surface. Although it cannot be ruled out that a single mixed phase is formed at temperatures higher than 110 K, we tentatively assign the α and β TPD features to desorption of water from bare and hydroxylated regions on the FeO film, respectively. Note also that the α feature only appears in the TPD spectra when a water coverage approximately twice the OH coverage is exceeded, indicating that the β feature corresponds to a phase incorporating a maximum H 2 O:OH ratio of 2:1, as is the case for the hexagonal ring structure discussed above. Alternatively, assignment of the α feature to a mixed phase, in which the OH groups are dispersed uniformly remains a possibility. However, this possibility appears less likely, since a shift in the α peak as a function of the OH:H 2 O ratio would be expected, which was barely observed. Note, however, that at the highest H 2 O coverages in the presence of OH groups, the α state includes two components, indicating that the OH groups do have some effect on the desorption kinetics, though the cause of this is not clear at present. As noted above, the β TPD feature, associated with water adsorption at OH groups, shifts to higher temperatures both with increasing H 2 O coverage and increasing OH coverage. The peak positions in the different experiments are plotted together in Fig. 5f , along with the positions of the α peak of the bare film for comparison. Variation in the β desorption temperature with OH coverage may reflect differences in H 2 O cluster size due to isolation of OH groups in separate moiré unit cells, since the number of OH groups per cell determines the maximum number of water molecules that can be stabilized in each. This is supported by comparison of the STM images shown in Fig. 6a,c , obtained on surfaces with the same quantity (0.1 ML) of water adsorbed onto FeO films with OH coverages of 0.12 and 0.05 ML, respectively. On the surface with the lower OH coverage ( Fig. 6c ), a large number of smaller clusters is observed, whereas on the surface with high OH coverage ( Fig. 6a ) a smaller number of larger clusters is seen. The corresponding difference in desorption temperature for these two systems is ~4 K ( Fig. 5f ). It is not clear from the present results whether these subtle effects, apparently due to cluster size, result from increasing thermodynamic stability with increasing size or from more complex kinetic factors. Finally, a feature of the TPD data worth noting is the invariance of the second-layer γ desorption temperature irrespective of the surface OH coverage ( Fig. 5a–e ). This result shows that the enhanced hydrophilicity conferred to the surface by the OH groups is lost after formation of the first H 2 O monolayer. This is similar to hydrophobic water layers studied previously on hydrophobic Pt(111) [49] and graphite [50] surfaces as well as on a hydrophilic kaolinite surface [51] . In all these cases, the preferential downward orientation of O–H bonds in the outermost water layers left surfaces devoid of ‘dangling H-bonds’ which could bind strongly to the next layer of water. Our TPD results thus provide further support for the ‘H-down’ model of the hexagonal water structure on the hydroxylated FeO film, and indicate that, in spite of the very weak interactions with the surface, the structure formed on the bare FeO surface likewise contains few or no H 2 O molecules with O–H bonds directed away from the surface. The broader implications of this result are not trivial; under ambient temperature conditions, thermal flipping of O–H bonds away from the surface can be sufficient to create hydrophilic interactions on a surface which is hydrophobic at low temperatures, as exemplified by recent MD simulations of water interacting with kaolinite [52] , [53] . Our STM, DFT and TPD studies addressing water clustering on bare and hydroxylated FeO surfaces reveal that highly localized hydrophilic domains are formed upon hydroxylation of a moiré-structured FeO monolayer on Pt(111), such that adsorbed water forms nanometre-sized clusters rather than extended two-dimensional islands. The water clusters exhibit a hexameric ring structure stabilized by hydrogen bonding with surface OH groups, in contrast to the larger islands on the bare surface which exhibit an amorphous structure. The STM and DFT results suggest that within the hexagonal structure, half of the water molecules accept H-bonds from surface OH groups while the other half donate H-bonds to surface O ions, resulting in an H 2 O:OH ratio of 2:1. This 2:1 ratio is supported by TPD measurements, which show a single desorption feature for H 2 O coverages up to approximately twice the initial OH coverage. Remarkably, when this ratio is exceeded, excess water adsorbed on the surface is neither incorporated into the hexagonal structure, forming a phase with a diluted OH concentration, nor is it induced to form an ordered structure by proximity with the hexagonal phase. Rather, by STM, we observe a coexistence of ordered and disordered water structures on a scale of 1 nm. This result highlights the very localized influence of OH groups on the structure of the adsorbed water monolayer, in contrast to what has been observed on metal surfaces, where only small concentrations of defects are sufficient to induce large-scale formation of ordered structures locked into simple registry with the substrate [4] . Detailed investigation, by DFT, of orientational ordering of water molecules in hexagonal H 2 O nanoclusters shows that cooperative hydrogen bonding effects play a substantial role in determining the details of the structures and the interactions between water molecules and the surface. Stronger molecule–surface interactions are found to compensate for weaker intermolecular interactions in certain structures—in one case through spontaneous formation of an H 3 O + ion—so that otherwise unfavourable configurations at the cluster edges are energetically comparable to the more balanced H-bond donor–acceptor configuration which is by far most stable in the gas phase. The discovered templating effect of the hydroxylated FeO film allows control of the dispersion of adsorbates, making it an intriguing surface for the study of small clusters of water and other hydrophilic species. It would be interesting to investigate the orientational ordering and proton transfer dynamics of H 2 O in few-molecule clusters at lower temperatures, where such structures can be fully or partially frozen. One can further envision using the hydroxylated FeO film to control the bottom-up synthesis of nanostructures based on hydrophilic components or precursors; though the templating effects of the bare FeO film itself are rather weak, being observed most clearly only at very low temperatures [23] , [24] , hydrogen bonding with surface OH groups should significantly enhance ordering, enabling directed self-assembly at higher temperatures. STM and TPD Measurements Monolayer FeO films were grown [20] , [54] by evaporation of Fe onto clean, sputtered and annealed Pt(111) surfaces followed by heating in 1 × 10 −6 mbar O 2 at 1,000 K. STM measurements were performed using a home-built variable-temperature Aarhus STM [55] , mounted in an ultra-high vacuum (UHV) chamber with a base pressure of ~1 × 10 −10 mbar. For STM experiments, water exposures were performed by removing the cooled sample ( T =110 K) from the STM block using the in-vacuum transfer arm so that the sample faced the water inlet. The tip of the transfer arm was pre-cooled by pressing it against the cold STM block for several minutes, and the dosing procedure was performed as quickly as possible (<1 min) to keep the sample temperature as low as possible (<135 K). Deionized water, degassed by several freeze-pump-thaw cycles, was dosed onto the surface using 1 ms pulses from a binary piezoelectric valve. Calibration of water coverages was performed by deposition onto clean Pt(111), where water forms an overlayer with known density [7] of 1.1 × 10 15 cm −2 . The surface coverage of 1 ML is defined here as the density of O atoms in the FeO film, 1.2 × 10 15 cm −2 . It was determined that a single pulse from the piezoelectric doser produced a water coverage of ~0.02 ML on the surface. Unless otherwise noted, STM images of water structures were acquired at +1.0–1.5 V sample bias and tunnelling currents of 0.1–0.2 nA. STM image processing was conducted using the Gwyddion software package [56] . TPD experiments were carried out using a commercial UHV surface analysis system (SPECS), equipped with a Hiden quadrupole mass spectrometer (QMS) fitted with a glass shroud with a 4-mm entrance aperture as well as an X-ray source and electron energy analyzer for X-ray photoelectron spectroscopy, a SPECS variable-temperature STM-150 (Aarhus), and similar equipment for sample preparation as on the home-built STM system. For these experiments, a hat-shaped Pt(111) crystal 7 mm in diameter was used, with a type K thermocouple spot-welded to the side of the crystal. Liquid nitrogen cooling allowed the sample to be cooled to ~110 K, and a filament placed behind the sample provided radiative and electron-beam heating up to ~1,200 K. Water was dosed at 130 K by backfilling the chamber with a leak valve and a Eurotherm temperature controller was used to provide the linear heating ramp for the TPD experiments, which was set at 2 K s −1 for all measurements. For experiments in both chambers, H atoms were produced from H 2 using thermal gas crackers and their coverage was determined by STM. Exposures were performed with the sample at room temperature, with the exception of the highest OH coverage (0.18ML), where the sample was held at 130 K to prevent reduction of the FeO film [28] . DFT Calculations All calculations were performed using the Vienna Ab initio Simulation Package [57] , [58] based on spin-polarized DFT. We used the DFT+U approach by Dudarev et al. [59] to correct the on-site Coulomb interaction between Fe 3 d orbitals. As in previous DFT studies of the FeO/Pt(111) system [30] , [60] , [61] we used the projector augmented wave method [62] , [63] and chose the parameters describing the on-site Coulomb interaction between Fe 3 d orbitals as U eff = U — J =3 eV. To model the 1 ML FeO/Pt(111) surface we used the experimentally observed (√91 × √91)R5.2° unit cell consisting of one layer of Fe atoms and one layer of O atoms supported on a three-layer Pt(111) slab. The FeO film, all adsorbates and the top Pt layer were fully relaxed, while the bottom two layers were fixed at bulk positions using the experimental value for the Pt–Pt spacing in the (111) plane of 2.77 Å (that is, an average Fe–Fe spacing of 3.09 Å). The Brillouin zone was sampled with the gamma point only. Exchange and correlation were described by the GGA-PW91 exchange-correlation functional [64] ; a kinetic energy cutoff of 400 eV was used. The initial guess for the magnetic structure is based on a row-wise anti-ferromagnetic structure, with a magnetic defect, due to the odd number of Fe atoms at the TOP domain [30] . How to cite this article: Merte, L. R. et al. Water clustering on nanostructured iron oxide films. Nat. Commun. 5:4193 doi: 10.1038/ncomms5193 (2014).